High-resolution optical spectroscopy using multimode interference in a compact tapered fibre Optical spectroscopy is a fundamental tool in numerous areas of science and technology. Much effort has focused on miniaturizing spectrometers, but thus far at the cost of spectral resolution and broad operating range. Here we describe a compact spectrometer that achieves both high spectral resolution and broad bandwidth. The device relies on imaging multimode interference from leaky modes along a multimode tapered optical fibre, resulting in spectrally distinguishable spatial patterns over a wide range of wavelengths from 500 to 1,600 nm. This tapered fibre multimode interference spectrometer achieves a spectral resolution down to 40 pm in the visible spectrum and 10 pm in the near-infrared spectrum (corresponding to resolving powers of 10 4 –10 5 ). Multimode interference spectroscopy is suitable in a variety of device geometries, including planar waveguides in a broad range of transparent materials. Since its nineteenth century origins with Walleston and Frauenhofer [1] , modern spectroscopy has become an essential tool for scientific research, including analytical chemistry, biochemical sensing [2] , [3] , material analysis [4] , optical communication [5] , [6] and medical applications [7] . Modern grating spectrometers project the spectral components of light onto a photodetector array, and some commercially available systems [8] , [9] , [10] , [11] are able to achieve very high resolving powers exceeding R> 10 6 as quantified by the resolving power, where δω is the spectral resolution at frequency ω 0 . However, high-resolution grating spectrometers are inevitably bulky because their spectral resolution scales inversely with optical path length. Fourier transform spectrometers can be more compact in size, but their scanning interferometric configuration makes them slow for large bandwidth applications. In recent years, there has been a strong effort to develop novel spectrometers that are compact and have high resolving powers and operational bandwidths [5] , [12] , [13] , [14] , [15] , [16] , [17] , [18] , [19] , [20] , [21] , [22] , [23] , [24] , [25] , [26] , [27] . In addition to miniature grating spectrometers [12] , resonant structures such as nanocavities [13] , [14] , [15] , [16] , [17] , [18] have also been employed to separate spectral components into unique detectors. This research has produced millimetre-scale spectrometers with high resolving powers of R >10 4 , but with limited fractional bandwidth, . Another class of compact spectrometers relies on imaging the speckle patterns of a photonic bandgap fibre bundle [19] or a multimode optical fibre [20] , [21] , [22] . However, these spectrometers are centimetres to metres long, which can result in the instability of the interference pattern due to environmental fluctuations, hence limiting their long-term operation. Recently, a silicon-based spectrometer [23] that measures the multimode transmission profile from a disordered photonic crystal structure achieved a resolving power comparable to typical grating spectrometers, but it requires coupling to a subwavelength input waveguide and has a limited bandwidth from 1,500 to 1,525 nm. A high-resolution Fourier transform spectrometer [24] has also been demonstrated on-chip, but its narrow free spectral range limits its operation bandwidth to 0.75 at 1,550 nm. Although some of these recently developed compact spectrometers can already match the spectral resolution of grating spectrometers, a compact device with both high resolving power and broad operating bandwidth remains elusive. Here we introduce a compact spectrometer based on multimode interference (MMI) that simultaneously achieves high resolving power of R >10 4 ( R >10 5 ) in the visible (near-infrared) spectrum, and bandwidth B ∼ 1 in a millimetre-scale device. 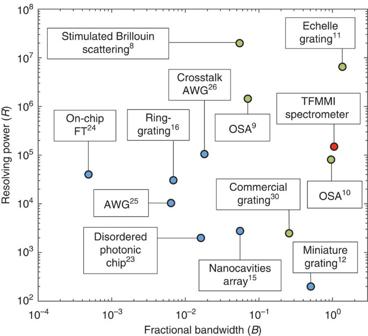Figure 1: Comparison of various compact and bench-top spectrometers. Various metrics can be used to compare compact spectrometers, two of which—the fractional bandwidth,Band resolving power,R—are compared in this figure. For the purpose of comparison, we also include five commercial bench-top spectrometers (green): optical spectrum analysers (OSA), a stimulated Brillouin scattering spectrometer, an Echelle spectrometer and a single-grating spectrometer (note that multi-grating spectrometers can have wider operating bandwidth). Shown in blue are some of the recently developed compact spectrometers. The TFMMI spectrometer (red) that is introduced in this work achieves a resolving power ofR>104(R>105) in the visible (near-infrared) spectrum, and bandwidthB∼1. AWG, arrayed waveguide grating, FT, Fourier transform spectrometer. Using MMI for spectroscopy Figure 1 compares the resolving powers and fractional bandwidth of several bench-top and compact spectrometers, including the device introduced in this work. Supplementary Table 1 provides more details about these spectrometers. The device is based on a tapered multimode fibre, as illustrated in Fig. 2a , produced by tapering a multimode optical fibre (Thorlabs AFS105/125y) using the flame-brush technique with taper lengths ∼ 5 mm. A non-adiabatic taper angle causes light at frequency ω to couple to a large number of spatial modes with different propagation constants, resulting in a unique interference profile that can be imaged as a ‘fingerprint’, or basis state, of a given frequency ω . Specifically, in the tapered optical fibre, the electric field varies in the propagation direction z as Figure 1: Comparison of various compact and bench-top spectrometers. Various metrics can be used to compare compact spectrometers, two of which—the fractional bandwidth, B and resolving power, R —are compared in this figure. For the purpose of comparison, we also include five commercial bench-top spectrometers (green): optical spectrum analysers (OSA), a stimulated Brillouin scattering spectrometer, an Echelle spectrometer and a single-grating spectrometer (note that multi-grating spectrometers can have wider operating bandwidth). Shown in blue are some of the recently developed compact spectrometers. The TFMMI spectrometer (red) that is introduced in this work achieves a resolving power of R >10 4 ( R >10 5 ) in the visible (near-infrared) spectrum, and bandwidth B ∼ 1. AWG, arrayed waveguide grating, FT, Fourier transform spectrometer. 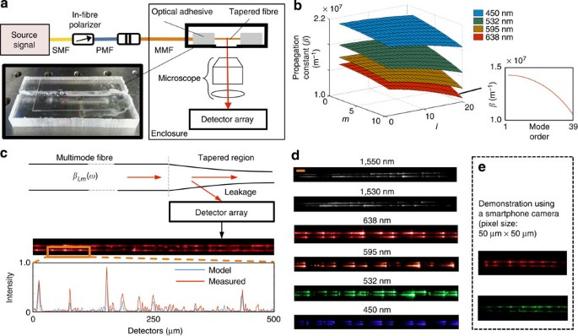Figure 2: Using MMI in a tapered fibre for optical spectroscopy. (a) Imaging set-up used in the experiment. The device is mounted securely in an acrylic holder using optical adhesives and is imaged through a cover glass. MMF, multimode fibre; PMF, polarization-maintaining fibre; SMF, single-mode fibre. (b) Isoplanes of propagation constants at four frequencies corresponding toλ=450, 532, 595 and 638nm for a silica fiber of core radius 30μm. Inset: propagation constant as a function of mode order. (c) Schematic of the TFMMI spectrometer, consisting of a tapered fibre imaged on a commercial camera. The optical image shows the device when a 638-nm laser was directed through the tapered fibre. The intensity distribution is extracted from one MMI section for the purpose of illustration, showing qualitative agreement between experiment and model. (d) Monochrome and optical images show the spatial intensity distribution for wavelengths of 1,550, 1,530, 638, 595, 532 and 450 nm monochromatic fields through the tapered fibre. Scale bar, 50 μm. (e) Imaging the fibre using a smartphone camera shows a potential for portable and field applications. Full size image Figure 2: Using MMI in a tapered fibre for optical spectroscopy. ( a ) Imaging set-up used in the experiment. The device is mounted securely in an acrylic holder using optical adhesives and is imaged through a cover glass. MMF, multimode fibre; PMF, polarization-maintaining fibre; SMF, single-mode fibre. ( b ) Isoplanes of propagation constants at four frequencies corresponding to λ =450, 532, 595 and 638nm for a silica fiber of core radius 30μm. Inset: propagation constant as a function of mode order. ( c ) Schematic of the TFMMI spectrometer, consisting of a tapered fibre imaged on a commercial camera. The optical image shows the device when a 638-nm laser was directed through the tapered fibre. The intensity distribution is extracted from one MMI section for the purpose of illustration, showing qualitative agreement between experiment and model. ( d ) Monochrome and optical images show the spatial intensity distribution for wavelengths of 1,550, 1,530, 638, 595, 532 and 450 nm monochromatic fields through the tapered fibre. Scale bar, 50 μm. ( e ) Imaging the fibre using a smartphone camera shows a potential for portable and field applications. Full size image where E l,m are the spatial profiles of the Bessel modes l and m in the fibre, φ l,m are the initial phase offsets, and β l,m (z) are the phase propagation constants, plotted in Fig. 2b . The tapering of the fibre leads to a non-uniform modal dispersion, which modifies the interference along the taper length, as reflected in the z -dependent propagation constant β l,m ( z ) and E l,m ( z ), while also changing the mode confinement, leading to radiative losses. Imaging of the far-field interference pattern I ( x , y , z , ω )=| E ( x , y , z , ω , t )| 2 and subsequent basis mapping enables resolving power in excess of R =10 5 and broad bandwidth B ∼ 1. This tapered fibre MMI (TFMMI) imaging approach enables unique performance compared with other spectroscopy tools ( Fig. 1 ). Characterization and spectroscopy scheme We coupled light into the TFMMI using a butt-coupled single-mode fibre with in-fibre polarizer (OZ Optics). This coupling was long-term stable and robust against coupling misalignment, mechanical vibrations and polarization drifts, as will be described in the section below. We then characterized the device in a × 17 microscope set-up ( Fig. 2a ). For calibration, we acquired a series of images of 1.5 mm of the tapered region with a waist ranging from 30 to 10 μm in diameter while scanning a narrow linewidth (<10 MHz) laser from 634.800 to 639.400 nm in steps of 2 pm and from 1,500.000 to 1,580.000 nm in steps of 1 pm. Figure 2d shows examples of these calibration images at wavelengths of (638, 595, 532, 450) nm in the visible spectrum and (1,550, 1,530) nm in near-infrared. The images associated with each wavelength formed the column vectors in our calibration matrix that converts between spatial patterns and input frequencies. 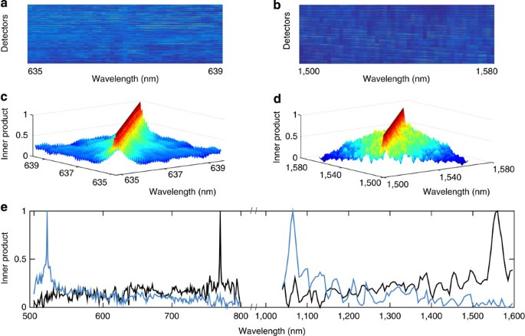Figure 3: Spectroscopy scheme. The frequency states corresponding to intensity images describe a spectral-to-spatial map. (a,b) Calibration matrix showing the intensity distributions of different wavelengths through the fibre from 634.800 to 639.400 nm and from 1,500.000 to 1,580.000 nm. (c,d) Monotonically decreasing inner products showing decreasing overlap of spatial distribution of the matrix inaandb, respectively. (e) The inner products between wavelengths from 500 to 800 nm and from 1,040 to 1,595 nm decay, showing that no two distinguishable wavelengths have the same associated fingerprint. Figure 3a,b shows the resulting calibration matrices for visible and near-infrared wavelengths, respectively. Equation (1) predicts that different colours produce distinguishable camera images in the limit of a very long tapered fibre. The finite pixel size of the camera and fibre length, and the number of imaged modes could result in basis images that may not be fully orthogonal. To verify that the images (column vectors) are distinguishable, we evaluated their cross-correlation by computing every permutation of the inner product between two different wavelengths vector and : for an ideal TFMMI of long length, and for all i≠j after normalization. In practice, there is background noise and crosstalk between these states due to the finite length of the fibre, but as seen from Fig. 3c,d , the inner products monotonically decrease to an isolation level of ∼ 10 −1 as the wavelength separation increases. Figure 3: Spectroscopy scheme. The frequency states corresponding to intensity images describe a spectral-to-spatial map. ( a , b ) Calibration matrix showing the intensity distributions of different wavelengths through the fibre from 634.800 to 639.400 nm and from 1,500.000 to 1,580.000 nm. ( c , d ) Monotonically decreasing inner products showing decreasing overlap of spatial distribution of the matrix in a and b , respectively. ( e ) The inner products between wavelengths from 500 to 800 nm and from 1,040 to 1,595 nm decay, showing that no two distinguishable wavelengths have the same associated fingerprint. Full size image In principle, the TFMMI spectrometer supports a broad wavelength range from 400 nm up to 2,400 nm due to the broad transparency window of silica fibre [28] . However, we did not have the instruments to test this full range. Instead, we used a monochromator (Acton SP2500) and a supercontinuum source (NKT SuperK Extreme) to produce a 1-nm wide probe signal to extend our previous analysis to 500 nm< λ< 800 nm and 1,100 nm< λ <1,600 nm. Figure 3e indicates a nearly orthonormal basis set at these wavelengths. To resolve an arbitrary input, the signal’s spectrum is related by to the detected MMI patterns , where Λ is the calibration matrix. Matrix left-inversion gives a least-square solution , which applies in situations even when where are the calibrated frequencies, that is, the spectral reconstruction works even for a continuous input spectrum. In addition, this solution can be treated as an initial solution to the more general minimization problem where ||·|| 2 denotes the 2-norm [19] , [20] , [21] , [22] , [23] , [29] . By eliminating the non-physical negative solutions and then solving this minimization problem using a nonlinear optimization algorithm, we can reconstruct the spectra of a measured signal more accurately (see Supplementary Methods for further discussion). Experimental results On the basis of the spectroscopy scheme discussed in the previous section, we used our TFMMI spectrometer to reconstruct the spectra of multiple probe beams. 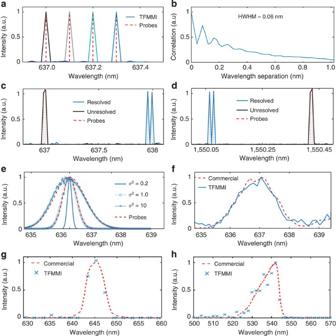Figure 4: Performance of the TFMMI spectrometer. In all the following reconstructions, no assumptions on the nature of the light signal were madea priori. (a) On the basis of the spectroscopy scheme discussed above, we used our TFMMI spectrometer to reconstruct multiple narrow spectra. (b) Spectral correlation function shows a half-width at half-maximum ofδλ≈ 0.06 nm. (c) We verified the resolution by directly resolving two closely spaced spectral components using our constructed spectrometer. Sharply peaked input wavelengths of 637.96 and 638.00 nm are clearly resolved, while input wavelengths of 637.00 and 637.02 nm are not fully resolved, bounding the resolution to 40 pm at 638 nm. (d) Sharply peaked input wavelengths of 1,550.070 and 1,550.080 nm are clearly resolved while input wavelengths of 1,550.410 and 1,550.415 nm are not fully resolved; thus the resolution of the device is bounded to 10 pm at 1,550 nm. (e) Reconstruction of Gaussian spectra with different variances. (f) Reconstructed spectrum of a continuous signal showing good agreement with that obtained with a commercial spectrometer. (g,h) The spectrometer was also able to reconstruct more broadband signals with spectral components from 640 to 655 nm and 520 to 550 nm. Figure 4a shows the successful reconstruction of four laser lines (red dashed line) using our constructed spectrometer (coloured solid lines). Figure 4: Performance of the TFMMI spectrometer. In all the following reconstructions, no assumptions on the nature of the light signal were made a priori . ( a ) On the basis of the spectroscopy scheme discussed above, we used our TFMMI spectrometer to reconstruct multiple narrow spectra. ( b ) Spectral correlation function shows a half-width at half-maximum of δλ ≈ 0.06 nm. ( c ) We verified the resolution by directly resolving two closely spaced spectral components using our constructed spectrometer. Sharply peaked input wavelengths of 637.96 and 638.00 nm are clearly resolved, while input wavelengths of 637.00 and 637.02 nm are not fully resolved, bounding the resolution to 40 pm at 638 nm. ( d ) Sharply peaked input wavelengths of 1,550.070 and 1,550.080 nm are clearly resolved while input wavelengths of 1,550.410 and 1,550.415 nm are not fully resolved; thus the resolution of the device is bounded to 10 pm at 1,550 nm. ( e ) Reconstruction of Gaussian spectra with different variances. ( f ) Reconstructed spectrum of a continuous signal showing good agreement with that obtained with a commercial spectrometer. ( g , h ) The spectrometer was also able to reconstruct more broadband signals with spectral components from 640 to 655 nm and 520 to 550 nm. Full size image We can estimate the spectral resolution of the device from a correlation function [20] , [21] , [22] , [23] C ( δλ,m )=〈 u ( λ,m ) u ( λ+δλ,m )〉 λ /[〈 u ( λ,m )〉 λ 〈 u ( λ+δλ,m )〉 λ ]−1 where u ( λ,m ) is the intensity of pixel m for image vector of wavelength λ. The average correlation over all pixels was normalized as shown in Fig. 4b . The half-width at half-maximum of δλ ≈0.06 nm approximates the spectral resolution, that is, wavelength vectors that are approximately separated by 0.06 nm at λ ≈637 nm are sufficiently distinguishable. We directly determined the spectral resolution of the TFMMI spectrometer by measuring the intensity profiles of two nearby input wavelengths at various power levels. Images were acquired sequentially and summed to produce the addition of two frequency states. Over tens-of-milliseconds integration times of these experiments, there would be no interference between these laser fields given that they are separated by more than 1 pm (0.7 GHz) at 637 nm. Therefore, adding sequential measurements at different frequencies is justified (though twice the readout noise is introduced compared with a single exposure). The detuning between the pair of wavelengths was gradually increased to find the wavelength separation at which the reconstruction algorithm could resolve them. This is the case at Δ λ =40 pm in the visible regime ( Fig. 4c ) and Δ λ =10 pm in the ΝIR regime ( Fig. 4d ), providing the upper bounds of the TFMMI resolution in these spectral ranges. Using the same device and calibration matrix, we reconstructed multiple narrow laser lines as shown in Fig. 4a and multiple broader synthesized Gaussian spectra ( Fig. 4e ). In Fig. 4f–h , we demonstrate that the device can reconstruct continuous spectra in a single exposure. In Fig. 4f , we measured a 2-nm bandwidth (full-width at half-maximum) input signal generated by filtering a supercontinuum light source (NKT SuperK Extreme). The red dashed line shows a measurement on a commercial grating spectrometer [30] , which matches closely the reconstructed spectrum from the TFMMI device. In Fig. 4g,h , we extend the input bandwidth to 10 and 15 nm, respectively. For this measurement, we calibrated the fibre spectrometer using an acousto-optic tunable filter in steps of 2 nm (filter bandwidth of 2 nm). We find good agreement with the measured spectra at 10-nm bandwidth ( Fig. 4h ) and qualitative agreement at 15-nm bandwidth ( Fig. 4g ). Long-term stability and repeatability It is also important to evaluate the long-term stability of the TFMMI spectrometer, as interference-based devices can be sensitive to changing environmental conditions. To minimize the susceptibility of this spectrometer to mechanical vibrations, we securely mounted the tapered fibre in an acrylic fixture with a cover slip window. The calibration matrix obtained at a time interval of Δ t =(5 min, 12 h, 48 h) has an average correlation of (0.9977, 0.9835, 0.9588), indicating the long-term stability of the calibration. The decrease in correlation with time was primarily due to drifts in the three-axis stages; when the device was repositioned in the focal plane of the microscope, the correlation increased back to >0.98. Furthermore, the devices did not show noticeable degradation in performance over the maximum tested time of 4 months. The multimode section of the device is also sensitive to the spatial profile and polarization of the input mode. The spectrometer operates on the principle that the relative amplitudes of the excited MMF modes remain unchanged throughout the experiment. The single-mode input fibre with in-fibre polarizer provides high stability and repeatability—after 10 cycles of disconnecting and reconnecting the input channel with a monochromatic laser, the correlation between images, , was 0.9955±0.0034, indicating that the constructed device was insensitive to fibre alignment and input polarization. In addition, changes in temperature would alter the refractive index of the silica fibre. From the thermo-optic effect and equation (1), one can see that small temperature variation Δ T causes an offset ω → ω +Δ ω in the calibration and therefore affects the accuracy but not the precision of the reconstructed spectrum. In particular, the device would be insusceptible to temperature fluctuations if Δ T <(d n /d T R ) −1 ∼ 5 °C where n is the refractive index and d n /d T is the thermo-optic coefficient. Recent research [21] on the transverse speckle patterns in multimode fibres additionally indicates that the ∼ 15-cm-long fibre used in our experiment would remain correlated up to Δ T ∼ 10 °C. A shift of Δ ω may be applied [22] to correct the calibration for temperature variations >Δ T , and active thermal stabilization could also be implemented in applications where high spectral accuracy is needed in the presence of large ambient temperature changes. An important factor in a spectrometer is the photon detection efficiency. In our device, <1% of incident photons are detected because the leakage out of the tapered fibre is weak as 70–80% of input light remains guided in the fibre, and we only imaged 20–30% of the tapered region ( Supplementary Methods ). Various methods can be used to improve the collection efficiency. For example, optimizing the tapering parameters of the fibre or depositing nanoscatterers [31] could enhance the detection. A spiralled fibre geometry would increase the fraction of the fibre taper that is imaged on the camera. Imaging a longer section of fibre would also likely increase the spectral resolution. We have shown that the TFMMI device operates across a large spectral range from 500 to 1,600 nm and can precisely resolve sparse spectra, that is, spectra with few frequency components. For very broadband inputs, for example, spanning many tens of terahertz, the contrast of the interference fringes diminishes, resulting in lower signal-to-noise and worse frequency reconstruction. Improving the spatial resolution of the microscope imaging would improve the interference visibility. In addition, dispersion engineering in the tapered fibre could be used to produce distinguishable wavelength patterns for targeted spectral signatures across a broad spectrum. The fibre configuration suggests that the TFMMI spectrometer would be most suitable in fibre-coupled applications in which signals could be efficiently channelled to a single-mode input fibre. Although the device was not optimized for any specific figures of merit, the spectrometer’s narrow spectral resolution of 40 pm (10 pm)—corresponding to resolving powers of 15,950 (155,000) at 635 nm (1,550 nm)—and broad operational range from 500 to 1,600 nm show unique advantages of the MMF-based spectroscopy approach. The millimetre-scale size of our device is already comparable to those of recent compact spectrometers ( Supplementary Table 1 ) and could be reduced further by directly integrating the detector arrays with the tapered optical fibre. Furthermore, the TFMMI spectrometer concept can be realized in a variety of on-chip configurations and materials, including tapered waveguides for the ultraviolet and mid-IR spectral ranges. Optimized geometries, such as on-chip tapered waveguide spirals, will likely allow for improved photon collection efficiency. Such compact spectrometers based on MMI in tapered fibres or in on-chip waveguides promise picometer-class spectroscopy in lab-on-a-chip and portable applications. How to cite this article: Wan, N. H. et al . High-resolution optical spectroscopy using multimode interference in a compact tapered fibre. Nat. Commun. 6:7762 doi: 10.1038/ncomms8762 (2015).